Profiling lymphocyte interactions at the single-cell level by microfluidic cell pairing Establishing a successful immune response requires cell–cell interactions, where the nature of antigen presentation dictates functional outcomes. Methods to study these interactions, however, suffer from limited throughput and a lack of control over cell pairing. Here we describe a microfluidic platform that achieves high-throughput deterministic pairing of lymphocytes with a defined contact time, thereby allowing accurate assessment of early activation events for each pair in controlled microenvironments. More importantly, the platform allows the capture of dynamic processes and static parameters from both partners simultaneously, thus enabling pairwise-correlated multiparametric profiling of lymphocyte interactions over hundreds of pairs in a single experiment. Using our platform, we characterized early activation dynamics of CD8 T cells (OT-1 and TRP1 transnuclear (TN)) and investigated the extent of heterogeneity in T-cell activation and the correlation of multiple readouts. The results establish our platform as a promising tool for quantitative investigation of lymphocyte interactions. Adaptive immune responses begin with interactions of lymphocytes and antigen-presenting cells (APCs). Engagement of immunoreceptors together with co-stimulatory and co-inhibitory molecules serves as the initial stage towards fate diversity. Although the identities of the molecules involved in these interactions are known [1] , [2] , [3] , a comprehensive understanding of underlying molecular mechanisms necessitates a more dynamic visualization of these interactions. Technical advances such as intravital multiphoton microscopy [4] , [5] , [6] , [7] , [8] , [9] , reporter mice [10] , [11] , [12] and synthetic signal transduction pathways [13] , [14] have enabled some of these analyses in vivo , but the complexity and lack of control of the in vivo microenvironment makes it challenging to fully tease out causal factors in these interactions. This in turn motivates the development of complementary in vitro platforms to study lymphocyte activation in a controlled environment with real-time imaging and adequate numbers of cells for meaningful statistical analysis. Cell–cell interactions are usually studied by initiating contact via brief centrifugal co-sedimentation, followed by analysis using flow cytometry of cell pairs [15] , [16] , [17] . In this setting, the interactions between cells are neither controlled nor well-defined (for example, number of interacting partners, duration of cell–cell contacts and so on). Flow cytometry also precludes investigation of temporal dynamics within a single-cell pair. Alternative approaches include immobilization of one of the interacting partners on poly- L -lysine-coated cover slips and then adding the second partner from the top [18] , [19] , [20] , [21] , [22] , [23] . Although these studies have provided key insights into immune cell activation, this approach has limited throughput and does not provide adequate control over pairing (for example, timing of interactions, movement of partner cells, duration of contacts and so on), thus complicating analysis and interpretation of results. Use of supported planar bilayers provide a more controlled approach, yet this technique does not recapitulate the complete physiology of APCs [24] , [25] . Critically, no approach tracks the interacting partners over time while maintaining control of the microenvironment to allow sequential probing of individual cell pairs, thus precluding the ability to acquire cell correlated multiparametric phenotypic data across a large number of cell pairs. To address these shortcomings, we developed a microfluidic platform to trap and controllably pair hundreds of lymphocytes, using a deterministic cell-loading protocol based on passive hydrodynamics. The platform achieves requisite control over pairings with one-to-one interacting partners, well-defined and synchronous initiation of interactions and enduring contacts. We can thus examine the early interaction dynamics of lymphocytes in a controlled manner. It provides full control of the soluble microenvironment by media exchange without losing cell registration. This feature enables sequential probing of cell pairs through on-chip stimulation, staining and fixation protocols. Using our devices, we demonstrate dynamic pairwise profiling of interactions between CD8 T cells and APCs at the single-pair level and perform measurements on both partners. We further used our devices to characterize the early activation dynamics of CD8 T cells from two melanoma-specific TN mouse models, which recognize the identical antigen with vastly different affinities [26] . We observed that the differences in T-cell receptor (TCR) affinity for pMHCI (peptides bound to major histocompatibility complex class I glycoprotein) complex result in qualitatively and quantitatively different T-cell activation kinetics. These, in turn, correlate with differential output of cytokines. Together, our data establish the microfluidic cell pairing platform as a valuable tool for investigation of cell–cell interactions in immunology. Microfluidic device design and characterization We developed the microfluidic devices by adopting design principles from our work on stem cell reprogramming via fusion [27] . As immune cells are considerably smaller (~3 × ) and more deformable than stem cells, and because of the lithographic limitations and nonlinear scaling of fluid flow that accompany a reduction in dimensions, we altered the device design and geometries for use with primary lymphocytes. Devices contain a dense array of weir-based silicone (polydimethylsiloxane, PDMS) hydrodynamic cell traps in a flow-through channel ( Fig. 1a,b ). Each cell trap consists of a back-side single-cell capture cup and a front-side two-cell capture cup. Support pillars on each side of the capture cups allow fluid flow through the cups to direct cells into traps and are made slightly shorter than the cell diameter for cell capture. To maximize the pairing efficiency with minimal clogging, we optimized the trap designs to increase the ratio of fractional fluid flow through the cups versus around the cups by altering the column spacings, row spacings, capture cup widths and spacings between support pillars. We chose the largest possible spacing between support pillars to increase the flow through the cups without compromising the number of traps that can be placed in a row. In addition, we chose the smallest possible column spacing to reduce the flow around the cups with minimal clogging. The selection of these two parameters had the most prominent effect on pairing efficiencies. Capture cup widths were tailored based on the size of the immune cells, and made slightly larger than mean cell size to accommodate variation. Row spacings had the most dominant effect on cell clogging and were chosen to allow for efficient loading to minimize aggregate formation. We found that column spacings of 7–9 μm, row spacings of 12–16 μm, cup widths of 8–10 μm and 10–12 μm spacing between support pillars were optimal for maximum cell pairing efficiencies. To account for the deformability of immune cells, we set the support pillar height to total height ratio to 0.2–0.25 to prevent cells from squeezing under the traps. 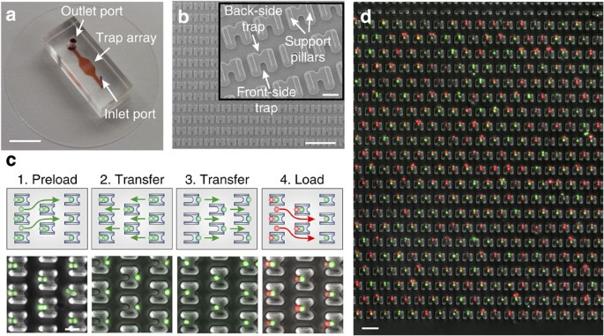Figure 1: Microfluidic device for immune cell pairing. (a) Image of the microfluidic cell pairing device. Channels and trap array are in red. (b) Scanning electron micrograph image of the cell trap array showing the back-side single-cell traps, front-side two-cell traps and support pillars. (c) Four-step cell-loading and pairing protocol. The first cell population (green cells) is preloaded into the front-side traps until the device is saturated (first step). This step enables use of 1–5 μl of cell solutions by directly pipetting on the inlet reservoir. The direction of the flow is reversed to load the cells into the back-side single-cell traps (second step). The additional cells flow around the cups and are flushed out of the device. The direction of flow is reversed once again to transfer the cells into the larger front-side two-cell traps two rows below (third step). Finally, the second cell population (red cells) is loaded and cells are captured in the front-side traps right in front of the first cell type (fourth step). (d) Overlaid phase contrast and fluorescence images showing primary mouse lymphocytes stained with DiI (red) and DiO (green) membrane dyes paired in the traps. Scale bars: (a) 5 mm, (b) 100 μm, 20 μm (inset), (c) 20 μm, (d) 50 μm. Figure 1: Microfluidic device for immune cell pairing. ( a ) Image of the microfluidic cell pairing device. Channels and trap array are in red. ( b ) Scanning electron micrograph image of the cell trap array showing the back-side single-cell traps, front-side two-cell traps and support pillars. ( c ) Four-step cell-loading and pairing protocol. The first cell population (green cells) is preloaded into the front-side traps until the device is saturated (first step). This step enables use of 1–5 μl of cell solutions by directly pipetting on the inlet reservoir. The direction of the flow is reversed to load the cells into the back-side single-cell traps (second step). The additional cells flow around the cups and are flushed out of the device. The direction of flow is reversed once again to transfer the cells into the larger front-side two-cell traps two rows below (third step). Finally, the second cell population (red cells) is loaded and cells are captured in the front-side traps right in front of the first cell type (fourth step). ( d ) Overlaid phase contrast and fluorescence images showing primary mouse lymphocytes stained with DiI (red) and DiO (green) membrane dyes paired in the traps. Scale bars: ( a ) 5 mm, ( b ) 100 μm, 20 μm (inset), ( c ) 20 μm, ( d ) 50 μm. Full size image With reduction in device dimensions (spacing between cups, channel height), fluidic resistance in the device increases nonlinearly and limits the operational range of pressures and flow rates along with switching time of flow direction. Our cell-loading protocol requires the flow direction to be reversed promptly to enable efficient cell pairing. We therefore determined the maximal length of the cell capture array (hence, the total number of traps in the device) for minimal fluidic resistance to allow fast fluid switching with practical flow rates provided by standard syringe pumps. We evaluated the ability of our devices to properly capture and pair immune cells using primary lymphocytes. With optimized device geometries, we could capture up to ~80% of cells that entered the array and obtain fill factors of >95% (percentage of traps correctly occupied; trap density: 500–850 traps per mm 2 ). We achieved cell pairing efficiencies between 40 and 85% (mean 67±12%; n =18) using a four-step back-and-forth loading procedure ( Fig. 1c,d ). Cell loading and pairing was sample efficient (~10 4 cells) and fast, with <40 s delay across the device. Once pairing was achieved, cells were actively held paired and in contact by maintaining a slight forward flow, which also enabled exchange of solutions without losing the pairing and registration of cells in the array. Monitoring early events during lymphocyte activation We demonstrated the utility of our devices in monitoring of early activation dynamics of lymphocytes by measurement of cytosolic Ca 2+ mobilization of CD8 T cells—a rapid and sensitive readout of TCR engagement [28] , [29] . We used Fura-2-loaded CD8 T cells from TCR transgenic OT-I mice [30] , which recognize the ovalbumin-derived peptide SIINFEKL (corresponding to amino-acid residues 257–264; OVA 257–264 ) bound to the major histocompatibility complex (MHC) class I (MHCI) allele H-2K b , and used primary CD40-activated B cells as APCs ( Supplementary Movie 1 ). We recorded from hundreds of T cells at once in a single experiment without the need for pooling data from multiple runs, and observe heterogeneity in cellular responses upon stimulation via chemicals (ionomycin), antibody-coated beads and APCs ( Fig. 2 ). By pairing T cells with APCs loaded with serial dilutions of antigen, we generated dose-response profiles and quantitatively analysed their responses ( Fig. 3 , Supplementary Fig. 1 ). Increasing concentrations of antigen increased the percentage of responding cells ( Fig. 3a,c , Supplementary Fig. 1a,c and Supplementary Table 1 ), similar to that observed in parallel bulk assays, using upregulation of CD25 as readout ( Supplementary Fig. 2 ). Higher antigen concentrations also increased integrated Ca 2+ levels and reduced delays in onset and peak times ( Fig. 3c , Supplementary Fig. 1c ). We further run unsupervised statistical clustering algorithms on the responses to identify distinct patterns ( Fig. 3b , Supplementary Fig. 1b ). We observed considerable cell-to-cell variation in the dynamics of the Ca 2+ response, which became more prominent with decreasing antigen concentrations, as inferred from the differences in integrated Ca 2+ levels and onset times of the clusters. Cells responded more uniformly at high antigen concentrations, suggesting that monocolonal populations of CD8 T cells behave in relatively homogenous manner but only upon activation with strong stimuli ( Fig. 3b , Supplementary Fig. 1b and Supplementary Table 1 ). We also recorded dose-response curves using chemical stimulants, where the cells were captured in single-cell trap mode and activated using serial dilutions of ionomycin ( Supplementary Fig. 3a ). We observed the expected dose-dependent activation ( Supplementary Fig. 3b ), demonstrating that T cells on-chip behave similar to that in conventional systems. 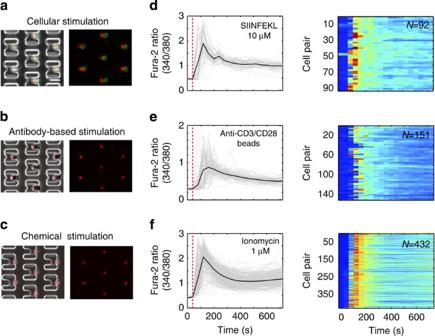Figure 2: Activation of OT-I CD8 T cells through different modes of stimulation and imaging of cytosolic Ca2+mobilization. (a) Stimulation of T cells through antigen presentation by antigenic peptide loaded B cells. Fura-2-stained T cells are shown in false colour (red). B cells express eGFP-labelled MHCII, shown in green. (b) Stimulation of T cells (false colour, red) through pairing with anti-CD3/CD28 antibody-coated beads. (c) Stimulation of T cells (false colour, red) through chemical agents (ionomycin). Cells are trapped in the back-side single-cell traps, and ionomycin solution is flowed over the cells during the course of experiment. (d–f) Time plots (left) showing the calcium signalling profiles of OT-1 CD8 T cells upon (d) antigen presentation, (e) bead-based stimulation and (f) ionomycin stimulation. Each grey trace represents the response of a single T cell. Black traces represent the average responses. Corresponding heat maps are shown to the right, each row corresponding to the calcium response (Fura-2 ratio) of an individual cell where blue indicates low calcium, red indicates high. Range for heat maps is the same as their corresponding time plots to the left.Nrepresents the number of cells for which the responses are shown. Scale bar, 10 μm, shown only inaapplies to all images shown ina–c. Red dotted lines in the time plots ofd–findicate the pairing times, that is, the time T cells make contact with B cells (a) or beads (b). Red dotted line in time plot ofcrepresents the stimulation time of T cells with ionomycin. Figure 2: Activation of OT-I CD8 T cells through different modes of stimulation and imaging of cytosolic Ca 2+ mobilization. ( a ) Stimulation of T cells through antigen presentation by antigenic peptide loaded B cells. Fura-2-stained T cells are shown in false colour (red). B cells express eGFP-labelled MHCII, shown in green. ( b ) Stimulation of T cells (false colour, red) through pairing with anti-CD3/CD28 antibody-coated beads. ( c ) Stimulation of T cells (false colour, red) through chemical agents (ionomycin). Cells are trapped in the back-side single-cell traps, and ionomycin solution is flowed over the cells during the course of experiment. ( d – f ) Time plots (left) showing the calcium signalling profiles of OT-1 CD8 T cells upon ( d ) antigen presentation, ( e ) bead-based stimulation and ( f ) ionomycin stimulation. Each grey trace represents the response of a single T cell. Black traces represent the average responses. Corresponding heat maps are shown to the right, each row corresponding to the calcium response (Fura-2 ratio) of an individual cell where blue indicates low calcium, red indicates high. Range for heat maps is the same as their corresponding time plots to the left. N represents the number of cells for which the responses are shown. Scale bar, 10 μm, shown only in a applies to all images shown in a – c . Red dotted lines in the time plots of d – f indicate the pairing times, that is, the time T cells make contact with B cells ( a ) or beads ( b ). Red dotted line in time plot of c represents the stimulation time of T cells with ionomycin. 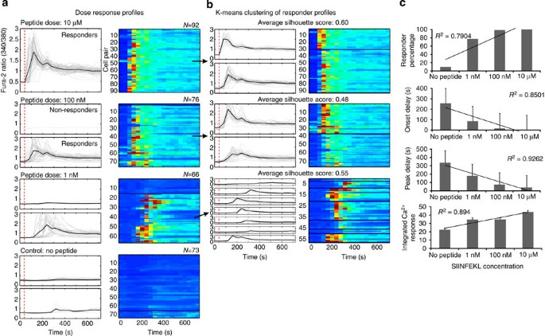Figure 3: Monitoring early activation dynamics of OT-I CD8 T cells. (a) Responder (bottom panels) and non-responder (top panels) signalling profiles with corresponding heat maps for serial dilutions of SIINFEKL peptide loaded onto B-cell APCs. (b) K-means clustering of responder cells showing that the heterogeneity between clusters are increasing with lower doses inferred from increased variation in onset times, calcium waveforms and number of clusters. For each peptide dose ina, corresponding cluster plots for responder cells were shown on the right inbindicated by black arrows. (c) Bar graphs showing the trends in responder percentages, onset and peak delays, and integrated Ca2+response of OT-I CD8 T cells with increasing peptide concentration. Linear fits shown with coefficient of determination (R2); linear trends are significantP<0.05. Error bars represent the s.d. of single-cell responses. For heat maps ina,b, each line corresponds to the calcium response (Fura-2 ratio) of an individual cell where blue indicates low calcium, red indicates high. Range for heat maps is the same as their corresponding time plots to the left: 0 (low)–3 (high). Red dotted lines indicate the pairing times. Results are representative of three independent experiments. Full size image Figure 3: Monitoring early activation dynamics of OT-I CD8 T cells. ( a ) Responder (bottom panels) and non-responder (top panels) signalling profiles with corresponding heat maps for serial dilutions of SIINFEKL peptide loaded onto B-cell APCs. ( b ) K-means clustering of responder cells showing that the heterogeneity between clusters are increasing with lower doses inferred from increased variation in onset times, calcium waveforms and number of clusters. For each peptide dose in a , corresponding cluster plots for responder cells were shown on the right in b indicated by black arrows. ( c ) Bar graphs showing the trends in responder percentages, onset and peak delays, and integrated Ca 2+ response of OT-I CD8 T cells with increasing peptide concentration. Linear fits shown with coefficient of determination ( R 2 ); linear trends are significant P <0.05. Error bars represent the s.d. of single-cell responses. For heat maps in a , b , each line corresponds to the calcium response (Fura-2 ratio) of an individual cell where blue indicates low calcium, red indicates high. Range for heat maps is the same as their corresponding time plots to the left: 0 (low)–3 (high). Red dotted lines indicate the pairing times. Results are representative of three independent experiments. Full size image Next, we evaluated the feasibility of our devices to assay the early molecular events during lymphocyte activation. Upon stimulation, the information from the engaged membrane receptors are communicated to their nuclear or cytoplasmic targets via signalling molecules. Number and dynamics of their phosphorylation states regulate downstream processes. As a demonstration, we measured phosphorylation of extracellular signal-regulated kinase (ERK), a central component of the TCR signalling pathway that coordinates a wide range of responses including proliferation, differentiation and survival [31] , [32] . We stimulated CD8 T cells by pairing them with anti-CD3/CD28 antibody-coated beads in the same manner as with cells and recorded their Ca 2+ mobilization. We then fixed the cells on-chip 200 s after pairing, and measured their ERK phosphorylation (ppERK) levels by on-chip staining and imaging ( Fig. 4a,b ). We observed that, under the conditions used, less than half of the cells responded to antibody stimulation within the 200-s time window as inferred from Ca 2+ mobilization, and responder cells exhibited a wide distribution in their integrated Ca 2+ magnitudes, onset times and ppERK levels ( Fig. 4c ). Observation of single-cell responses revealed that the ppERK levels showed an increase with shorter onset times and higher integrated Ca 2+ levels ( Supplementary Fig. 4a ). However, because of the heterogeneous nature of these responses, the pairwise trends can be approximated only by a weak linear relationship. To resolve the patterns more explicitly, we also included the temporal evolution of calcium profiles in our analysis, and performed unsupervised clustering on calcium dynamics together with its correlation to ppERK levels ( Fig. 4d ). Our analysis organized responder cells into distinct clusters, and based on the responses of these clusters we found that higher ppERK levels were correlated with shorter onset times and higher integrated Ca 2+ levels ( P <0.05) as expected ( Fig. 4e and Supplementary Fig. 4b,c ). The Ca 2+ signalling and ppERK levels of the non-responder cells were similar to control (unpaired) cells ( P >0.1; Supplementary Fig. 4d ) verifying that these cells did not show activation within the experimental time frame. 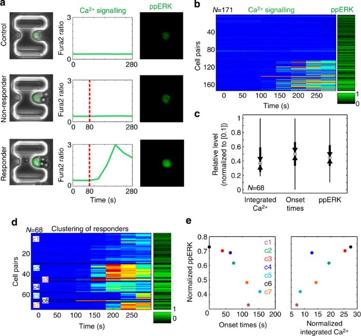Figure 4: Measurement of early molecular events of OT-I CD8 T-cell activation. (a) Cells were stimulated with anti-CD3/CD28 antibody-coated beads, and cytosolic Ca2+levels were recorded. Cells were fixed 200 s after stimulation with beads, and ERK phosphorylation levels were measured by on-chip staining and imaging cytometry. Red dotted lines indicate the pairing times of T cells with the beads. Cells with increased Ca2+activity displayed higher ppERK levels. (b) Heat map showing the calcium and ppERK responses of OT-I CD8 cells. Only 68 of the 171 cells responded to antibody stimulation within the 200-s time window. (c) Box plot of integrated calcium, onset times and ppERK levels showing their distribution. All values are normalized to [0, 1]. The black dot inside white circle represents the median, the upper and lower edges of the box represents the upper and lower quartiles, The triangles represent theP<0.05 significance interval. The whiskers represent the outliers within 1.5 times the interquartile range. (d) K-means clustering of responder profiles indicating seven clusters with distinct calcium waveforms. Clusters are separated with a black line, and labelled with c1-c7 for identification. (e) Plots showing the correlation of ppERK levels to onset times and integrated Ca2+levels (P<0.05). Clusters are represented using different colours as indicated (that is, c3–cluster3 shown in red). For heat maps inbandd, the range for calcium traces is from 0 (low) to 3 (high) where blue indicates low calcium, red indicates high. Results are representative of two independent experiments. Significant differences determined with one-way analysis of variance test. Figure 4: Measurement of early molecular events of OT-I CD8 T-cell activation. ( a ) Cells were stimulated with anti-CD3/CD28 antibody-coated beads, and cytosolic Ca 2+ levels were recorded. Cells were fixed 200 s after stimulation with beads, and ERK phosphorylation levels were measured by on-chip staining and imaging cytometry. Red dotted lines indicate the pairing times of T cells with the beads. Cells with increased Ca 2+ activity displayed higher ppERK levels. ( b ) Heat map showing the calcium and ppERK responses of OT-I CD8 cells. Only 68 of the 171 cells responded to antibody stimulation within the 200-s time window. ( c ) Box plot of integrated calcium, onset times and ppERK levels showing their distribution. All values are normalized to [0, 1]. The black dot inside white circle represents the median, the upper and lower edges of the box represents the upper and lower quartiles, The triangles represent the P <0.05 significance interval. The whiskers represent the outliers within 1.5 times the interquartile range. ( d ) K-means clustering of responder profiles indicating seven clusters with distinct calcium waveforms. Clusters are separated with a black line, and labelled with c1-c7 for identification. ( e ) Plots showing the correlation of ppERK levels to onset times and integrated Ca 2+ levels ( P <0.05). Clusters are represented using different colours as indicated (that is, c3–cluster3 shown in red). For heat maps in b and d , the range for calcium traces is from 0 (low) to 3 (high) where blue indicates low calcium, red indicates high. Results are representative of two independent experiments. Significant differences determined with one-way analysis of variance test. Full size image In conventional assays, such phosphorylation measurements are generally performed after stimulating cells with brief co-sedimentation with APCs or beads, and fixing them after a certain time period [15] , [33] . This approach assumes homogeneous activation of cells and obscures the timing information. In addition, correlation analyses are generally performed by collecting measurements from independent assays using different aliquots of the same sample, and yield only average measures at the population level and not for the same cell. Our approach allows co-measurement and correlation of dynamic and static cell responses for each individual cell in a single straightforward assay with enhanced precision. Our results represent the first example of dynamic calcium measurements together with ERK phosphorylation for the same cells, and explicitly shows the correlation of ppERK levels not only to magnitude but also to the dynamics of the calcium signalling. These results demonstrate the efficiency of our platform for monitoring early events of lymphocyte activation in a controlled manner and at single-cell resolution. Pairwise profiling of lymphocyte interactions The ability to immobilize cell pairs within their traps and exchange solutions affords two unique opportunities for measurement. First, interacting partners can be imaged simultaneously and dynamic measurements can be performed for both partners in a pairwise-correlated manner. Second, once paired, partner cells can be further interrogated for their cellular markers by repeated on-chip staining and imaging. These capabilities allow pairwise and multiparametric profiling of lymphocytes during their interactions. To illustrate the power of this functionality, we studied the interaction between OT-I CD8 T cells and SIINFEKL-loaded MHCII-eGFP B cells. B cells were activated one day before experiments with anti-CD40 to increase their antigen presentation capability and upregulate co-stimulatory surface molecules. We first monitored cytosolic Ca 2+ mobilization for both partners during their engagement ( Fig. 5a ). Both T and B cells responded with an increase in cytosolic Ca 2+ within1 min after pairing, which took the form of the well-known peak-plateau-type calcium profile in most cell pairs. Then, by sequential antibody staining and imaging steps, we assayed for CD8 co-receptor surface expression on T cells and SIINFEKL-loaded MHCI (pMHCI) on B cells to measure the amount of antigen presented ( Fig. 5a ). We also measured MHCII-eGFP surface expression on B cells as a proxy for activation of B cells. We could then construct a detailed profile of the T cell–APC interactions by compiling and analysing the dynamic and static measurements together ( Fig. 5b ). 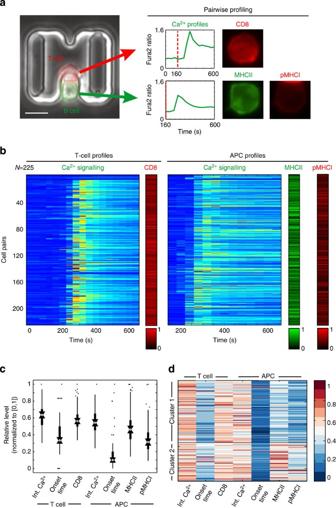Figure 5: Pairwise profiling of lymphocyte interactions. (a) Multiparametric data set obtained from the interacting partners through time-lapse microscopy, on-chip staining and imaging cytometry. (b) Interaction profiles of OT-I CD8 T cell–APCs compiled over 225 pairs showing the raw data set including calcium mobilization and the expression of CD8 (T cell), MHCII (APC) and pMHCI (APC) surface molecules. The cell pair responses were arranged based on T-cell calcium responses, that is, non-responders versus responders. The response profiles corresponding to non-responder T cells are separated from responder ones using a black line. Range for calcium heat maps: 0 (low)—2.5 (high) where blue indicates low calcium, red indicates high. (c) Box plots indicating the distribution of measured parameters over cell pairs. All values are normalized to [0, 1]. The black dot inside white circle represents the median, the upper and lower edges of the box represents the upper and lower quartiles, The triangles represent theP<0.05 significance interval. The whiskers represent the outliers within 1.5 times the interquartile range. Outliers beyond this range are indicated by *. (d) K-means clustering of interaction profiles. Clusters statistically differ in MHCII and pMHCI expression as determined by quantitative statistical comparison. Results are representative of three independent experiments. Figure 5: Pairwise profiling of lymphocyte interactions. ( a ) Multiparametric data set obtained from the interacting partners through time-lapse microscopy, on-chip staining and imaging cytometry. ( b ) Interaction profiles of OT-I CD8 T cell–APCs compiled over 225 pairs showing the raw data set including calcium mobilization and the expression of CD8 (T cell), MHCII (APC) and pMHCI (APC) surface molecules. The cell pair responses were arranged based on T-cell calcium responses, that is, non-responders versus responders. The response profiles corresponding to non-responder T cells are separated from responder ones using a black line. Range for calcium heat maps: 0 (low)—2.5 (high) where blue indicates low calcium, red indicates high. ( c ) Box plots indicating the distribution of measured parameters over cell pairs. All values are normalized to [0, 1]. The black dot inside white circle represents the median, the upper and lower edges of the box represents the upper and lower quartiles, The triangles represent the P <0.05 significance interval. The whiskers represent the outliers within 1.5 times the interquartile range. Outliers beyond this range are indicated by *. ( d ) K-means clustering of interaction profiles. Clusters statistically differ in MHCII and pMHCI expression as determined by quantitative statistical comparison. Results are representative of three independent experiments. Full size image Although both cell partners displayed a wide variation in their integrated Ca 2+ responses, onset times and expression of surface markers ( Fig. 5c and Supplementary Fig. 5e ), pairwise linear correlation analysis did not reveal any substantial correlation of any two parameters ( R 2 <0.2). To resolve any patterns in the responses, we performed unsupervised statistical data clustering based on all measured responses and our analysis organized the cell pairs into two clusters. Quantitative comparison of the responses revealed that the two clusters significantly differed in MHCII and pMHCI expression ( P <0.01; Fig. 5d ). Moreover, the cluster with higher expression of MHCII also showed a higher level of pMHCI as well (normalized MHCII expression: Cluster1=0.39±0.11, Cluster2=0.62±0.17, P <0.01; normalized pMHCI expression: Cluster1=0.27±0.11, Cluster2=0.46±0.15, P <0.01). One explanation for this observation is that both MHCI and MHCII are coordinately regulated along with other co-stimulatory molecules (that is, CD80, CD86), thus increasing their antigen presentation potential, and that cluster2 could include the subpopulation of B cells that are more strongly activated with CD40 signalling [34] , [35] , [36] . We further performed the clustering excluding either the MHCII or pMHCI expression levels to examine the relative importance of each of these parameters on observed clusters. Although removing pHMCI did not appreciably change the clustering distribution, the exclusion of MHCII changed the clustering considerably with different distribution of cell pairs, suggesting that the clustering was more dependent on the MHCII levels compared with pMHCI ( Supplementary Fig. 6 and Supplementary Table 2 ). Surprisingly, T-cell Ca 2+ responses did not correlate with pMHCI nor MHCII levels, which is probably due to the compensating effect of the high peptide concentrations used [37] . We then analysed the dynamics of calcium signalling to identify the differences in calcium waveforms and their relationship with other measured parameters. We observed that both T and B cells clustered into distinct subgroups based on their Ca 2+ signalling that could be classified as strong and weak responders, based on peak and integrated calcium levels ( Supplementary Fig. 5c,d ). As these strong or weak responder profiles did not show a significant correlation ( P >0.1) with other traits measured on the same or partner cell, this suggests other cell-intrinsic and cell-extrinsic sources for the observed variation. Taken together, these experiments demonstrate the ability of our method to obtain a multiparametric (in this case, five-dimensional) data set that includes single-cell correlated dynamic and static measurements on both partners in a single experiment and to construct detailed cell–cell interaction profiles in a pairwise-correlated manner not previously possible using other available assay formats. These profiles can then be studied by statistical analysis to identify the contributions of cell-intrinsic and -extrinsic factors on the interactions and to classify subpopulations. Tracking cell response histories to sequential stimulation Besides on-chip staining and fixation, the ability to exchange solutions enables sequential stimulation of cell pairs using soluble signals, which allows studies on antigen presentation to lymphocytes in dynamic environments. Especially with respect to lymphocyte differentiation, understanding how cell fate decisions are shaped during antigen presentation by concentration, timing and duration of soluble inputs in changing environments could benefit from the present approach [38] . Traditional dish- or cover slip-based approaches are not suitable for these types of studies, as they cannot maintain enduring interactions and track cellular responses while manipulating environments. Using this functionality, we investigated the calcium mobilization patterns of OT-I CD8 T cells upon sequential stimulation. Even freshly isolated TCR transgenic T cells are usually assumed to behave as a homogeneous population, but whether this assumption is correct remains to be established. We first paired T cells with antigen-loaded B cells, and subsequently performed ionomycin stimulation. We used antigenic peptides with varying TCR affinities [39] , [40] (SIINFEKL>Q4>T4>G4) at 10 μM concentration to further investigate how T cells regulate and adapt their response patterns depending on their affinity for antigen. For all antigenic peptides used, we found that cells could be classified as double responders (DRs), which responded to both stimulations, single responders (SRs), which responded only to ionomycin stimulation but not to antigen presentation, and finally non-responders, which did not respond to either stimulation ( Fig. 6a ). Unsupervised clustering separated the DR into two distinct groups that we named strong and weak responders based on integrated Ca 2+ levels ( Fig. 6b ). Although strong responders preserved their higher Ca 2+ levels with follow-up stimulation, weak responders show lower Ca 2+ use for both stimulations. Such distinct strong and weak responder patterns were also observed among the SR cells (ionomycin only responders) where ~50–70% of the SR showed higher Ca 2+ utilization ( Fig. 6c ). By examining the distribution of these responders within each population, we observed that the percentage of DR increases (that is, % of SR decreases) with increasing TCR affinities, along with an increase in the percentages of strong DR ( Fig. 6d and Supplementary Table 3 ). The relative percentage of the strong DR remained relatively constant at ~35–40% (that is, strong DR/total DR) with T4, Q4 and SIINFEKL peptide indicating saturation after T4. Similarly, the relative percentages of the SR did not depend on affinity. Together, these findings suggest that, among a given clonal population, there are strong and weak responders, and that strong responders maintain their higher response profiles upon subsequent stimulation. At the population level, the responder profiles display a shift towards stronger DR patterns with increasing TCR affinities (that is, stronger stimulus). Overall, these experiments provide insight into how heterogeneity prevalent among clonal cells manifests itself in cellular responses at the single-cell and population level, and demonstrate the first example of tracking cell response dynamics at single-cell level upon sequential probing and assessing the differences in responder profiles. 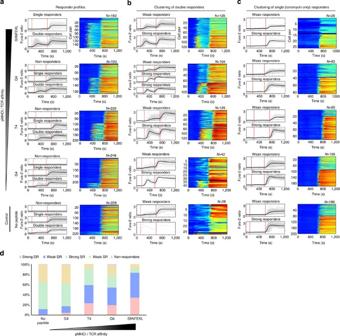Figure 6: Tracking OT-I CD8 T-cell response histories to sequential stimulation. (a) Cell response profiles to double stimulation. Cells were grouped as double responders (DRs), single responders (SRs) or non-responders. (b) Clustering of DR cells shown inainto strong and weak responders based on integrated Ca2+levels. For each peptide, clustering plots are shown to the right of their corresponding plots ina. (c) Clustering of SRs shown inainto strong and weak responders based on integrated Ca2+levels. (d) Distribution of responder types at the population level upon double stimulation with increasing pMHCI/TCR affinities. Range for heat maps ina–cis the same as their corresponding time plots to the left where blue indicates low calcium, red indicates high. The first red dotted line indicates the cell pairing time (antigen presentation), the second one marks ionomycin stimulation time.Nrepresents the number of cells for which the responses are shown. Results are representative of two independent experiments. Figure 6: Tracking OT-I CD8 T-cell response histories to sequential stimulation. ( a ) Cell response profiles to double stimulation. Cells were grouped as double responders (DRs), single responders (SRs) or non-responders. ( b ) Clustering of DR cells shown in a into strong and weak responders based on integrated Ca 2+ levels. For each peptide, clustering plots are shown to the right of their corresponding plots in a . ( c ) Clustering of SRs shown in a into strong and weak responders based on integrated Ca 2+ levels. ( d ) Distribution of responder types at the population level upon double stimulation with increasing pMHCI/TCR affinities. Range for heat maps in a – c is the same as their corresponding time plots to the left where blue indicates low calcium, red indicates high. The first red dotted line indicates the cell pairing time (antigen presentation), the second one marks ionomycin stimulation time. N represents the number of cells for which the responses are shown. Results are representative of two independent experiments. Full size image Early activation dynamics of TN TRP1 CD8 T cells We then applied our device to characterize the early activation dynamics of two lines of TN mice generated via somatic cell nuclear transfer [26] . CD8 T cells from both mice recognize the identical epitope derived from endogenous melanoma antigen TRP1 (tyrosinase-related protein 1, expressed in normal melanocytes and overexpressed in melanoma) but with tenfold different affinities as inferred from class I MHC tetramer dissociation. Despite the difference in their affinities, activated CD8 T cells from both high-affinity (TRP1 high ) and low-affinity (TRP1 low ) mice delayed the growth of melanoma in vivo to a similar extent [26] . Here we explored the implications of TCR affinity difference on their early activation dynamics. We paired CD8 T cells from TRP1 high and TRP1 low mice with CD40-activated B cells loaded with serial dilutions of a TRP1 heteroclitic variant peptide (peptide A1). TRP1 high T-cell populations exhibited strong Ca 2+ fluxes that had higher responder frequency, shorter delays in onset times and higher integrated Ca 2+ levels than those of TRP1 low cells ( Fig. 7a,b , Supplementary Fig. 7a and Supplementary Table 1 ). We also observed qualitative differences in the Ca 2+ waveforms. Although TRP1 high T cells exhibited a high transient peak followed by elevated steady-state Ca 2+ level, TRP1 low T cells showed incomplete/reduced signals where the peak was not generally present; instead Ca 2+ signalling was delayed, levels increased asymptotically and reached a plateau or decayed to baseline. However, in response to anti-CD3/CD28 antibody-coated beads, Ca 2+ signals in TRP1 low T cells were restored and were similar to those exhibited by TRP1 high T cells ( Fig. 7c , Supplementary Fig. 7b and Supplementary Table 1 ). We attribute this restoration of Ca 2+ signals to the much stronger engagement of the TCR signalling apparatus by antibodies than via the cognate pMHC. Overall, these results show that CD8 cells from two TN mice exhibit qualitatively and quantitatively distinct Ca 2+ responses along with considerable cell-to-cell variation within both T-cell populations. 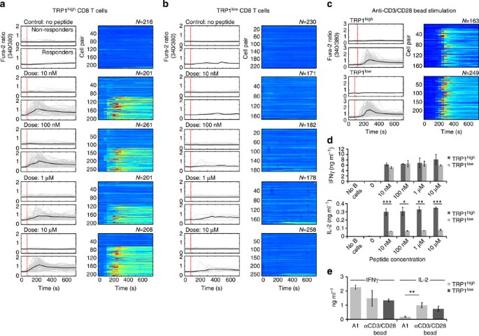Figure 7: Characterizing early activation dynamics in TRP1highand TRP1lowCD8 T cells. (a,b) Responder (bottom panels) and non-responder (top panels) signalling profiles of Trp1high(a) and Trp1low(b) CD8 T cells as determined by cytosolic Ca2+mobilization with corresponding heat maps for serial dilutions of TRP1 heteroclitic peptide A1. (c) Ca2+signals in TRP1 CD8 T cells in response to anti-CD3/CD28 bead stimulations. (a–c) Range for heat maps is the same as their corresponding time plots to the left. Red dotted lines indicate the pairing times.Nrepresents the number of cells for which the responses are shown. Results are representative of two independent experiments. (d) Cytokine secretion (IFNγ and IL-2) profiles for TRP1highand TRP1lowCD8 T cells assayed in bulk cultures run in parallel with microfluidic assay. (e) Cytokine secretion profiles for antibody bead stimulations. Results are representative of three independent experiments. Error bars represent the s.d. Significant differences determined with one-way analysis of variance test. *P<0.05; **P<0.01; ***P<0.001. Figure 7: Characterizing early activation dynamics in TRP1 high and TRP1 low CD8 T cells. ( a , b ) Responder (bottom panels) and non-responder (top panels) signalling profiles of Trp1 high ( a ) and Trp1 low ( b ) CD8 T cells as determined by cytosolic Ca 2+ mobilization with corresponding heat maps for serial dilutions of TRP1 heteroclitic peptide A1. ( c ) Ca 2+ signals in TRP1 CD8 T cells in response to anti-CD3/CD28 bead stimulations. ( a – c ) Range for heat maps is the same as their corresponding time plots to the left. Red dotted lines indicate the pairing times. N represents the number of cells for which the responses are shown. Results are representative of two independent experiments. ( d ) Cytokine secretion (IFNγ and IL-2) profiles for TRP1 high and TRP1 low CD8 T cells assayed in bulk cultures run in parallel with microfluidic assay. ( e ) Cytokine secretion profiles for antibody bead stimulations. Results are representative of three independent experiments. Error bars represent the s.d. Significant differences determined with one-way analysis of variance test. * P <0.05; ** P <0.01; *** P <0.001. Full size image Examining downstream cytokine production measured in bulk culture in parallel experiments, we found that while both TRP1 high and TRP1 low T cells produced similar amounts of interferon-γ (IFNγ; P >0.1), TRP1 high cells generated significantly higher quantities of interleukin-2 (IL-2; P <0.05, Fig. 7d ). Thus, although a peak-plateau response (high affinity) is correlated with both high IL-2 and IFNγ secretion, an atypical slow rise-plateau/decay response (low affinity) appears correlated with high IFNγ and low IL-2 secretion. In further support of this correlation, we found that the anti-CD3/CD28 antibody-coated beads that restored the peak-plateau Ca 2+ response in TRP1 low cells also recovered robust IL-2 and IFNγ production from TRP1 low cells ( P <0.01, Fig. 7e ). This establishes a link between TCR affinity and cytokine secretion patterns, and shows that low IL-2 secretion is not a limitation intrinsic to TRP1 low cells. These results are aligned with previous reports [16] , [19] , [41] , [42] and corroborate the hierarchy of cytokine secretion [43] , [44] and differential regulation by the dynamics of Ca 2+ signalling [45] , [46] . The affinity of TCR/pMHC interaction thus seems to determine the type of Ca 2+ signalling, which in turn helps set cytokine expression patterns. We further investigated the fine specificity of TCR/pMHC interactions using a panel of altered peptide ligands (APLs) generated by single amino-acid substitutions [26] . We performed our experiments on TRP1 high cells as they were more promiscuous in response to APLs than TRP1 low cells and exhibited differential cytokine expression. For peptide variants A1, K8, A3 and F8, TRP1 high T cells showed high responder frequencies with strong Ca 2+ fluxes, but with qualitative and quantitative differences in the response (onset delays, peak and integrated Ca 2+ levels; Fig. 8a , Supplementary Fig. 5c,d and Supplementary Table 3 ). These strong Ca 2+ signals were again correlated with high IFNγ and IL-2 secretion ( Fig. 8c ). For peptides A4, K4, and S8, responder percentages were lower, and signals were delayed and weak, similar to the responses of TRP1 low CD8 T cells to A1 peptide ( Fig. 8b , Supplementary Fig. 7c,d and Supplementary Table 4 ). As in TRP1 low cells, these weak Ca 2+ signals induced high levels of IFNγ but low levels of IL-2 ( Fig. 8c ). Only one peptide variant, E8, induced high responder frequency with weak Ca 2+ signals, but produced low levels of IL-2 ( Fig. 8b,c ). These data corroborate our earlier results that weak Ca 2+ signals induce low levels of IL-2, and show that this property is not limited to a particular TCR clonotype. 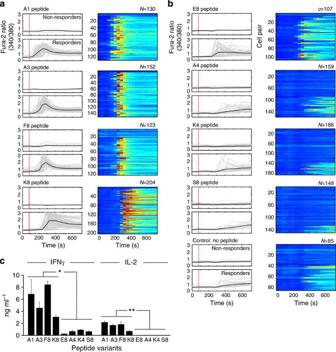Figure 8: Calcium signalling in TRP1highCD8 T cells in response to a set of altered peptide ligands. (a,b) TRP1highCD8 T cell Ca2+responses to peptide variants (a) A1, A3, F8 and K8, and (b) E8, A4, K4 and S8. (c) IFNγ and IL-2 production in TRP1highCD8 T cells in response to altered peptide ligands. Range for heat maps is the same as their corresponding time plots to the left: 0 (low)–3 (high). Red dotted lines indicate the pairing times.Nrepresents the number of cells for which the responses are shown. Results are representative of two independent experiments. Error bars represent s.d. Significant differences determined with one-way analysis of variance test. *P<0.05; **P<0.01. Figure 8: Calcium signalling in TRP1 high CD8 T cells in response to a set of altered peptide ligands. ( a , b ) TRP1 high CD8 T cell Ca 2+ responses to peptide variants ( a ) A1, A3, F8 and K8, and ( b ) E8, A4, K4 and S8. ( c ) IFNγ and IL-2 production in TRP1 high CD8 T cells in response to altered peptide ligands. Range for heat maps is the same as their corresponding time plots to the left: 0 (low)–3 (high). Red dotted lines indicate the pairing times. N represents the number of cells for which the responses are shown. Results are representative of two independent experiments. Error bars represent s.d. Significant differences determined with one-way analysis of variance test. * P <0.05; ** P <0.01. Full size image We developed a microfluidic cell pairing device for a comprehensive analysis of lymphocyte interactions in a well-defined and controlled setting. In comparison to conventional approaches, our platform offers several advantages. It provides control over pairings through one-to-one, enduring interactions with synchronous and precise timing of the contact initiation. Controlled pairing provides access to the earliest activation events from the exact moment of contact and in numbers required for statistical analysis (~100–200 cells in a single experiment at the required spatiotemporal resolution in this study). The ability to add reagents to cell pairs without losing track of them, as would occur in a bulk culture, enables application of temporally controlled soluble inputs. We can thus explore how different microenvironmental conditions affect immune cell priming and the ensuing activation cascade. The high efficiencies of cell capture and pairing would be especially beneficial when the available number of cells is insufficient for analysis using standard techniques such as flow cytometry. The presented approach should also be generally applicable to a wide range of cell types and sizes including the use of dendritic cells as APCs. Different cells would require re-optimization of the trap geometries and dimensions, which can readily be adapted to account for the different cell sizes and possible size mismatch for enabling successful pairing ( Supplementary Discussion ). Throughput can also be scaled up for applications that require the analysis of even larger number of cell pairs. We applied our platform to several experimental scenarios that would be technically challenging to perform using conventional methods. We assayed the early events of lymphocyte activation through imaging and cell fixation on-chip. This allowed analysis of single-cell heterogeneity with precise timings and quantifiable differences. Such data sets could especially benefit computational models for signalling cascades with refined single-cell data [15] , [33] , [47] , [48] . The ability to immobilize and preserve the pairs at defined locations within the array allowed us to obtain pairwise-correlated dynamic and static measurements over the interacting partners to inform on cell-intrinsic and cell-extrinsic factors on cellular responses observed subsequently [38] , [49] , [50] . By applying temporally controlled inputs, we could track cell histories in response to sequential stimuli and identify responder types among clonal populations. Finally, we used our device to examine early activation dynamics of CD8 T cells from two lines of melanoma-specific mouse models, each with different TCR affinities for cognate antigen. Differences in TCR affinities triggered different Ca 2+ mobilization dynamics and correlated with differential cytokine production. As determined through the use of a set of altered peptide ligands, the high TCR affinity induced strong Ca 2+ signals with robust IL-2 and IFNγ production, whereas low TCR affinity resulted in weak/reduced Ca 2+ spikes associated with high IFNγ and low IL-2 secretion. These data support the hierarchy of cytokine production based on TCR affinity [43] , [44] and are in agreement with the differential regulation of transcriptional activity, again correlated with different Ca 2+ dynamics [45] , [46] . The similarities and differences in cell responses observed here may have implications for in vivo behaviour of CD8 T cells. It could be that the early activation events are delayed for TRP1 low cells, and might occur with comparable efficiency by long-term engagement of antigens over the duration of complete immune response. Such long-term engagements have been suggested as a mechanism for fine-tuning the immune cell activation [41] , [51] . Similarly, increased IL-2 production from TRP1 high cells could preferentially recruit more T reg cells in the tumour microenvironment to depress their responses, or increased activation of the TRP1 high cells may be limiting their efficiency because of activation-induced cell death. In any case, the identification of exact mechanisms underlying how the differences in early dynamics are translated into similar functional outcomes warrants further investigation. The technique presented here can further be exploited and extended to other relevant studies in immunology including but not restricted to analysis of cell-mediated cytotoxicity, investigation of lymphocyte selection processes (that is, negative selection of immature B cells [52] , [53] ), asymmetric cell division upon antigen presentation [17] , [54] , [55] and correlation of early signalling with functional readout on longer time scales at the single-cell level. In conclusion, the microfluidic cell pairing device presents a useful approach for studying cell–cell interactions among lymphocytes and their interaction partners. It provides a complement to methodologies in biochemistry, genetics and high-resolution imaging through assessment of the dynamics of cellular responses instead of inferences based on snapshot analysis. In particular, we expect to be able to characterize the early events in lymphocyte activation and underlying mechanisms. It should also provide an additional tool to dissect out the contributions of cell-intrinsic (that is, T-cell parameters) and cell-extrinsic (that is, APC parameters, environment) factors on observed differentiation patterns and cell fate diversity upon activation. Animal care All animals were housed at the Whitehead Institute for Biomedical Research and were maintained according to the protocols approved by the MIT Committee on Animal Care. C57BL/6 and OT-I;RAG1 −/− transgenic mice were purchased from Jackson Labs. MHCII-eGFP mice [56] and TRP1 high and TRP1 low TN mice were generated in our lab [26] . Age 6- to 10-week-old mice of both sexes were used for experiments. Peptide production TRP1 altered peptide ligands were produced by Fmoc-based solid-phase peptide synthesis by the MIT Center for Cancer Research biopolymers facility. All peptides were dissolved in dimethyl sulfoxide (10 mg ml −1 ) and stored at −20 °C until further use. OVA peptides and variants were purchased from AnaSpec, EGT. Cell isolation, preparation and culture Cells were cultured in RPMI 1640 medium supplemented with 10% heat-inactivated FBS, 2 mM L -glutamine, 100 U ml −1 penicillin G sodium, 100 μg ml −1 streptomycin sulfate, 1 mM sodium pyruvate, 0.1 mM nonessential amino acids and 0.1 mM 2-Mercaptoethanol (2-ME). CD8 T cells were harvested from pooled spleen and lymph nodes of TRP1 high , TRP1 low or OT-I mice. Briefly, cell suspensions were subjected to hypotonic lysis to remove erythrocytes, filtered through a 40-μm cell strainer, and separated by positive selection on magnetic beads (Dynabeads, FlowComp Mouse CD8) according to the manufacturer’s instructions. For assessing pairing efficiencies ( Fig. 1d ), cells were stained with membrane dyes DiI and DiO (Life Technologies) following the manufacturer’s instructions. B cells were prepared from pooled spleen and lymph nodes of C57BL/6 or MHCII-eGFP mice using negative selection on magnetic beads (Miltenyi, B-cell isolation kit) according to the manufacturer’s instructions. Purified B cells were cultured in RPMI with anti-CD40 (BD, clone HM40–3, 1 μg ml −1 ) for 1 day before use. CD40-activated B cells were washed once in PBS, stained with 7-AAD (BD) viability dye, and live cells were sorted by FACS using an Aria II (BD) at the Whitehead Institute Flow Cytometry Core Facility. Sorted B cells were incubated at 37° with the indicated peptides for 30 min and washed twice with PBS before use. The identical T- and B-cell preparations were used for microfluidics assays and bulk culture assays that were run in parallel. For microfluidic assays, samples were treated with DNase (50 U ml −1 ; Ambion Turbo DNase, Life Technologies) to prevent long DNA segments from sticking in the device. For bulk culture, T cells and peptide-pulsed B cells were plated into round-bottom 96-well plates at a ratio of 100,000 T cells:100,000 B cells in 200 μl final volume RPMI. Supernatants were harvested at 24 or 72 h (from duplicate plates), as indicated and assayed for IL-2 or IFNγ by ELISA (BD). Co-culture cell pellets were stained with 7-AAD and antibodies to CD69, CD8, CD44 or CD25 following manufacturer protocols (all BD Pharmingen) as indicated to assess T-cell activation. Samples were analysed using a FACSCalibur (BD). Microfluidic device fabrication Masters for the microfluidic devices were fabricated using a two-layer SU-8 process. The first layer of photoresist (SU-8 2002, MicroChem) was spun at 10,00–1,500 r.p.m. for 30 s to yield feature heights of 2.2–3 μm. The wafers were exposed to ultraviolet light through a chrome mask (Advance Reproductions) to pattern the support pillars. After developing and baking, the second layer of photoresist (SU-8 2005) was spun at 1,000 r.p.m. for 30 s to yield feature heights of 7–9 μm. The wafers were then ultraviolet-exposed through a second chrome mask (Advance Reproductions) to generate cell trap patterns. Following developing and baking, SU-8 molds were hard-baked at 150 °C for 30 min, and were silanized for 2 h in a vacuum chamber saturated with Trichloromethylsilane (Sigma-Aldrich). We then made plastic masters as our final molds for future devices [57] . Devices were made by pouring PDMS over the master wafers followed by degassing and curing at 80 °C overnight. After curing, PDMS was peeled off, and individual devices were cut to proper sizes and holes for fluidic connections were punctured. To allow for integration with efficient ratiometric imaging, we plasma-bonded our devices to cover glasses of 0.17 mm thickness compatible with high numerical aperture (high-NA) fluorescence imaging. Microfluidic setup and cell-loading procedure Microfluidic devices were first filled with 70% ethanol and PBS to avoid generation of any bubbles. The surfaces were blocked using either 7.5% BSA or 10% pluronic F127 and incubating them at 37 °C for 1 h. The devices were then rinsed with media before assembly of fluidic connections and introduction of cells. Tygon Microbore tubing (Cole Parmer) connected to a four-way valve (UpChurch Scientific) was plugged into the outlet of the device. The valve was also connected to two 1 ml glass syringes (Hamilton) on two separate syringe pumps providing flow in opposite directions. Cells and reagents were pipetted directly into the inlet reservoir and withdrawn through the device. Cell loading and pairing was achieved using a four-step back-and-forth loading protocol ( Fig. 1c ). Initially, the device is preloaded by pipetting 1–5 μl of first cell population on the inlet reservoir and drawing into the device. This preloading step made it possible to use small numbers of cells within small volumes (10 6 –10 7 cells per ml, 1–5 μl aliquots) by eliminating cell loss due to dead spaces (syringe and tubing volumes) and avoiding settling of cells in stationary syringes. Once the device was saturated, the flow was reversed to isolate single cells in the back-side single-cell traps. When the extra cells were flushed out of the device, the inlet reservoir was washed by cell media and the flow was reversed again to transfer the cells in the opposing larger front-side two-cell traps. Finally, the second cell population is loaded on the inlet reservoir and withdrawn into the device to be trapped immediately in front of the previously trapped cells. During loading procedures, cell capture efficiencies, trap occupancies (fill factor) and loading times were calculated by taking into account the cell concentrations and sample volumes used. Cell capture efficiency is defined as the ratio of the number of cells being captured in traps to total cells entering the device. Fill factor is defined as the ratio of the number of traps occupied to total number of traps. Cell pairing efficiencies were dependent on cell-loading parameters (cell concentration, particular device dimension, loading times and flow rates) and also on inherent cell properties (cell stickiness and clumping, cell adhesion to surfaces, dead cell ratio and released DNA fragments, heterogeneity of the sample, that is, cell size, cell type). To minimize the influence of these factors, optimal loading conditions were determined for a given sample with preliminary trials, devices were blocked with BSA or pluronic F127, and cells were suspended in 1% BSA, 50 U ml −1 DNase solution and pipetted regularly to minimize cell adhesion and to keep cells homogenously distributed in the sample ( Supplementary Discussion ). Cell stimulation protocols Ionomycin stimulation was performed in single-cell trap mode, in which cells are trapped at the single-cell back-side capture traps and by perfusing ionomycin (Life Technologies) at various concentrations over trapped cells. Antibody stimulations were accomplished by pairing CD8 T cells with anti-CD3/CD28-coated microbeads (Life Technologies) in the same manner as in pairing with APCs. Because of the small size of the beads (4.5 μm) in comparison to cells, one T cell is generally paired with and stimulated by more than a single bead. For antigen presentation (cellular stimulations), primary mouse B cells were used as APCs, and cultured with anti-CD40 antibodies (Life Technologies) for 3 days before experiments. Anti-CD40-activated B cells were then incubated with serial dilutions of antigenic peptides at 37 °C for 30 min, washed with RPMI 1640 media to remove unbound peptide and resuspended in RPMI 1640 media supplemented with 10% FBS and 1% BSA before loading on chip to pair with T cells. Calcium imaging and analysis To monitor Ca 2+ signalling, cells were incubated in the dark with 1–3 μM Fura-2/AM (Life Technologies) ratiometric calcium indicator dye in serum-free RPMI 1640 (phenol red-free; Life Technologies) at 37 °C for 30 min. Cells were washed in RPMI 1640 by centrifugation and resuspended in RPMI 1640 supplemented with 10% FBS and 1% BSA for on-chip experiments. All experiments were conducted at room temperature (25 °C). Time-lapse imaging experiments were performed on an automated inverted microscope (Nikon Eclipse Ti, Nikon). For Ca 2+ imaging, exposure times were set while T cells were at rest and chosen close to saturation (but not saturated) when illuminated at 380 nm, and well below saturation when illuminated at 340 nm. Once set, exposure times were kept constant during all experiments. Images were acquired at × 20 magnification (S Plan Fluor ELWD 20x Ph1 ADM; Nikon) on a cooled CCD camera (CoolSNAP HQ 2 , Photometrics) using Nikon Elements Software (Nikon). Images were taken every 40 s from three to five fields of view and at each time point both phase and fluorescence images were acquired. Imaging was started when the T cells were trapped inside the front-side two-cell traps (when step 3 in Fig. 1c is completed), and a baseline measurement was taken before introducing the APCs (or beads). APCs were then introduced into the devices and pairing time was determined from the image frame where a T-cell appears in contact with an APC for the first time. The cell pairing was highly synchronous, and any remaining asynchronous pairing was measured and corrected during image analysis. Images were analysed in ImageJ ( http://rsb.info.nih.gov/ij/ ). Pairing efficiencies were calculated by determining the number of traps occupied by a single cell of one type paired with the second cell (or two) of the other type in all imaged field of views. For Ca 2+ measurements, region of interests (ROIs) were defined manually and chosen to cover the cell bodies. We verified that cells do not move out of ROIs during the course of the experiment. For T cells paired with more than a single APC, only T cells contacting one APC were included in the analysis. Fluorescent intensities for selected ROIs were exported as MS Excel (Microsoft) file for further analysis. Signals were analysed in Matlab (MathWorks) by custom written scripts. Time-lapse Ca 2+ signals were obtained by the ratio of fluorescence emission intensities at wavelengths 340 and 380 nm after background subtraction. The contact point was defined as time point corresponding to the phase image, in which the cell pair first appeared. As the criterion for activation, we used Ca 2+ increases greater than three standard deviations from the resting Ca 2+ level. ‘Ca 2+ onset time’ was taken as the time point before highest rise in the Ca 2+ trace or the time point of initial 20% increase from the baseline. ‘Onset delay’ was calculated by subtracting the contact time from onset time. ‘Peak delay’ was calculated by subtracting the contact time from the time point at which maximum Ca 2+ level was observed. Integrated Ca 2+ levels were calculated by integrating the Fura-2 ratio traces and normalizing to resting Ca 2+ levels. On-chip antibody staining, fixation and imaging cytometry Antibody staining was performed on chip by adapting the manufacturer’s protocols. The staining solutions were prepared at recommended dilutions in staining buffer (1 × PBS with 1% BSA), and flowed over the cells for recommended incubation durations (between 10 min and 2 h). Cell pairs were then washed with staining buffer before imaging. Cells were fixed on chip by flowing in 10% neutral buffered formalin for 10 min, washed with staining buffer and then permeabilized with 0.5% Triton X-100 for an additional 10 min. Cells were washed again with staining buffer before introducing antibody stains. For on-chip cytometry, cells were imaged at corresponding wavelengths, and intensity levels were recorded. For each stain, intensities were normalized within a range of 0 and 1, and data for calcium imaging and antibody stainings were matched for each cell and their interaction partner to construct their interaction profiles. Following antibodies were used in our assays: CD8 (BD Pharmingen), 25-D1.16 for OVA257–264 bound to H-2Kb (eBioscience), D13.14.4E for ppERK (Cell Signaling). Statistical analysis Unsupervised statistical clustering, either by k-means or one-dimensional hierarchical clustering algorithms, was performed in MATLAB on the multidimensional data set assembled using custom written scripts to resolve distinct classes of responders. For the k-means algorithm, sqEuclidean distance was used as the distance measure, and the number of clusters and quality of clustering were determined by optimizing over the average silhouette scores, which measures the dissimilarity of a point to its assigned cluster in comparison to other clusters. For hierarchical clustering, euclidean distance metric was used with ‘average’ as the linkage method. The clustering was optimized using assessing the cophenet scores. Principal component analysis was also performed to monitor the distribution of clusters. A two-tailed unpaired Student’s t -test was used to compare two samples. Multiple samples were compared using one-way analysis of variance test. Correction for multiple testing was made by using Tukey’s method. Statistical analyses were conducted using GraphPad Prism 6 (GraphPad Software). All data are reported as mean±s.d. How to cite this article: Dura, B. et al. Profiling lymphocyte interactions at the single-cell level by microfluidic cell pairing. Nat. Commun. 6:5940 doi: 10.1038/ncomms6940 (2015).